HHEX is a transcriptional regulator of the VEGFC/FLT4/PROX1 signaling axis during vascular development Formation of the lymphatic system requires the coordinated expression of several key regulators: vascular endothelial growth factor C (VEGFC), its receptor FLT4, and a key transcriptional effector, PROX1. Yet, how expression of these signaling components is regulated remains poorly understood. Here, using a combination of genetic and molecular approaches, we identify the transcription factor hematopoietically expressed homeobox (HHEX) as an upstream regulator of VEGFC , FLT4 , and PROX1 during angiogenic sprouting and lymphatic formation in vertebrates. By analyzing zebrafish mutants, we found that hhex is necessary for sprouting angiogenesis from the posterior cardinal vein, a process required for lymphangiogenesis. Furthermore, studies of mammalian HHEX using tissue-specific genetic deletions in mouse and knockdowns in cultured human endothelial cells reveal its highly conserved function during vascular and lymphatic development. Our findings that HHEX is essential for the regulation of the VEGFC/FLT4/PROX1 axis provide insights into the molecular regulation of lymphangiogenesis. Transcriptional regulation of endothelial cell fate and behavior is key to shape and maintain a competent vascular network. During development, lymphatic endothelial cells (LECs) have been reported to arise from a specific subset of vein endothelial cells and require the VEGFC/FLT4/PROX1 signaling axis for their migration, proliferation, and differentiation [1] , [2] , [3] . However, how the expression of these signaling components is regulated remains poorly understood. Of the transcription factor genes regulating endothelial cell physiology, hematopoietically expressed homeobox ( hhex ), also known as proline rich homeodomain ( prh ), is one of the earliest expressed by endothelial and hematopoietic precursors in frogs [4] , zebrafish [5] , and mice [6] . In zebrafish, Hhex can positively regulate endothelial and blood cell differentiation [5] ; however, analysis of a deletion allele which lacks hhex , as well as several other genes, suggests that Hhex is not essential for early endothelial and blood cell differentiation [5] . In mouse, Hhex mutants have multiple developmental defects including marked abnormalities in heart, liver, thyroid, and vascular formation [7] , [8] . In human endothelial and leukemic cells, HHEX is known to be a direct transcriptional regulator of VEGFA , VEGFR1 , and VEGFR2 [9] . However, its precise function during angiogenesis and lymphangiogenesis remains unclear. Through TAL effector nuclease (TALEN) mutagenesis, gene expression analysis, transplantation experiments and endothelial-specific overexpression, we show that in zebrafish, Hhex functions cell-autonomously in endothelial cells to regulate sprouting angiogenesis from the posterior cardinal vein (PCV) and subsequent lymphangiogenesis. We further show through knockdown experiments in vitro and genetic deletions in vivo that this crucial role during angiogenesis and lymphangiogenesis is conserved in mammals. Overall, our data show that HHEX controls blood vessel and lymphatic vessel formation by regulating the VEGFC/FLT4/PROX1 signaling axis. Zebrafish hhex mutants exhibit sprouting defects from the PCV HHEX is a transcription factor composed of a proline-rich domain and a highly conserved homeodomain [10] . Previously, we used the γ-ray-induced deletion allele b16 to investigate hhex function in zebrafish [10] . However, the b16 deletion affects the lower telomeric region of chromosome 12 and removes hhex and cyclops ( ndr2 ) as well as at least 14 other genes [11] . b16 mutants display pleiotropic phenotypes including cyclopia and curvature of the body axis [12] . Therefore, in order to determine more precisely the function of Hhex during zebrafish development, we generated hhex mutants using TALENs [13] . TALEN pairs were designed against the homeodomain sequence (Fig. 1a ) and two different alleles were recovered: hhex s721 which carries a 10 bp insertion leading to a premature stop codon and hhex s722 , an in-frame deletion of three amino acids (R149 to A151) in the second helix of the DNA-binding domain important for the stability of the protein during its interaction with DNA [14] (Fig. 1b ). In all our assays, both alleles exhibit the same phenotype. Fig. 1 Zebrafish hhex mutants lack sprouting angiogenesis from the posterior cardinal vein. a Schematic representation of Hhex. Hhex, 228 amino acids (aa) long, is composed of a proline-rich domain (4–113 aa) and a homeodomain (116–175 aa). b Alignment of partial Hhex homeodomain sequence in wild-type (WT), and two mutant alleles, hhex s721 and hhex s722 . The hhex s721 allele contains a 10 bp insertion leading to a premature stop codon within the homeodomain coding region, whereas the hhex s722 allele lacks amino acids R149 to A151. c , d Trunk vasculature of Tg(−5.2lyve1b:DsRed) ; hhex +/+ and hhex −/− embryos at 48 hpf. hhex mutant trunks exhibit a defect in sprouting angiogenesis from the posterior cardinal vein (PCV) (arrowheads point to tip cells sprouting from the PCV; asterisks indicate lack of tip cells sprouting from the PCV). e , f Trunk vasculature of Tg(−5.2lyve1b:DsRed) ; hhex +/+ and hhex −/− larvae at 5 dpf. hhex mutant trunks exhibit a defect in the formation of the venous intersegmental vessels (vISVs), the thoracic duct (TD) lymphatic vessel, and the dorsal longitudinal lymphatic vessel (DLLV) (arrowhead points to a vISV; arrows point to the ventrally positioned TD and dorsally positioned DLLV; asterisks indicate lack of these structures). g , h Brightfield lateral views of hhex +/+ and hhex −/− larvae at 5 dpf. Mutant larvae exhibit pericardial edema (arrowhead). Scale bars: 100 μm Full size image In the zebrafish axial vasculature, sprouting angiogenesis occurs in two waves. Sprouting from the dorsal aorta starts at 20 hours post fertilization (hpf) to give rise to arterial intersegmental vessels (aISVs) [15] . Subsequently, endothelial sprouting from the PCV occurs between 32 and 36 hpf [15] and this process gives rise to both venous ISVs (vISVs) and LECs [16] . aISVs appear to form normally in hhex mutants (Supplementary Fig. 1c, d ); however, using the Tg(−5.2lyve1b:DsRed) line to visualize the venous and lymphatics endothelial cells, we observed that hhex mutants lack most sprouting vessels from the PCV (Fig. 1c, d ). Time-lapse imaging of wild-type and mutant embryos show that while sprouting angiogenesis from the PCV is clearly observed in wild-type siblings between 32 and 36 hpf, no cell migration from the PCV is visible in hhex mutants at least until 48 hpf (Supplementary Movies 1 , 2 ). Furthermore, at 5 days post fertilization (dpf), hhex mutants exhibit pericardial edema (Fig. 1g, h ), a near absence of vISVs, a complete loss of trunk lymphatic vessels, and a strong reduction of facial lymphatic vessels (Fig. 1e, f , Supplementary Fig. 1e–i , Supplementary Fig. 2 ). Altogether, these observations indicate that Hhex regulates the earliest step of sprouting angiogenesis and lymphangiogenesis from the PCV. Vegfc/Flt4/Prox1 signaling axis is affected in hhex mutants Angiogenesis is mostly regulated by vascular endothelial growth factors (VEGFs) and their receptors (VEGFRs). Similar to hhex mutants, vegfc and flt4 (also known as vegfr3 ) mutants also fail to initiate sprouting angiogenesis and lymphangiogenesis from the PCV [16] , [17] , [18] , [19] . Additionally, hhex mutants exhibit a delayed formation of the primordial hindbrain channels at 26 hpf (Supplementary Fig. 1a, b ), similar to vegfc and flt4 mutants [17] , [18] . Therefore, we decided to examine the Vegfc/Flt4 signaling pathway in hhex mutants. We first assessed vegfc and flt4 expression at 24 and 32 hpf by whole-mount in situ hybridization (Fig. 2a–h ). At 24 hpf, hhex mutants exhibit decreased flt4 expression while vegfc was slightly increased and ectopically expressed in the PCV (Fig. 2a–d ). These changes were more pronounced at 32 hpf, as flt4 expression was greatly decreased in hhex mutants, whereas vegfc expression in the PCV was clearly increased (Fig. 2e–h ). To test whether the phenotype we observed in hhex mutants might at least in part be due to the modulation of the Vegfc/Flt4 signaling pathway, we performed a rescue experiment by injecting messenger RNA (mRNA) encoding full-length human FLT4 as previously used in zebrafish [18] . Confocal imaging of the trunk vasculature of hhex mutant larvae and quantification of vISVs and thoracic duct (TD) extensions revealed a partial rescue of vISVs and lymphatic formation after FLT4 mRNA injection (Fig. 2i–l ), indicating that the Vegfc/Flt4 signaling pathway functions downstream of Hhex. Altogether, these results show that Hhex is a crucial regulator of both flt4 and vegfc expression in the PCV during angiogenic sprouting. Fig. 2 The Vegfc/Flt4 pathway is affected in zebrafish hhex mutants. a – d Whole-mount in situ hybridization showing flt4 ( a , b ) and vegfc ( c , d ) expression in 24 hpf hhex +/+ and hhex −/− embryos. At 24 hpf, hhex mutants exhibit decreased flt4 expression (asterisks), whereas vegfc expression in the PCV appears to be slightly increased (arrowheads). e – h Whole-mount in situ hybridization showing flt4 ( e , f ) and vegfc ( g , h ) expression at 32 hpf in hhex +/+ and hhex −/− embryos. At 32 hpf, hhex mutants exhibit a strong decrease in flt4 expression (asterisks), whereas vegfc expression is clearly increased in the PCV (arrowheads). x / y : number of embryos showing representative phenotype ( x ), number of embryos examined ( y ). i Trunk vasculature of 5 dpf Tg(kdrl:EGFP); hhex −/− injected, or not, with full-length human FLT4 mRNA. hhex mutants exhibit partial rescue of their vISVs at 5 dpf (arrowheads point to vISVs). j Quantification of vISVs across 10 somites in 5 dpf non-injected hhex −/− ( n = 6) and FLT4 mRNA-injected hhex −/− ( n = 8). k Trunk lymphatic vasculature of 5 dpf Tg(−5.2lyve1b:DsRed); hhex −/− injected, or not, with full-length human FLT4 mRNA. hhex mutants exhibit partial rescue of their TD at 5 dpf (arrowheads point to vISVs and arrow points to TD). l Quantification of TD extensions across 10 somites in 5 dpf non-injected hhex −/− ( n = 6) and FLT4 mRNA-injected hhex −/− ( n = 7). Values represent means ± s.e.m. **** P ≤ 0.0001 and * P ≤ 0.05 by t -test. Scale bars: 50 μm Full size image In addition to its role in blood vessel development, the VEGFC/FLT4 signaling axis also plays an instructive role during lymphatic vessel development via activation of the transcription factor PROX1 [20] , [21] . Given that hhex mutants display strongly reduced lymphatic formation, we sought to determine whether lymphatic specification was affected in hhex mutants by immunostaining for Prox1. In wild-type siblings at 36 hpf, Prox1 + endothelial cells are observed in the dorsal part of the PCV. In contrast, hhex mutants show a near absence of Prox1 + endothelial cells in the dorsal part of the PCV, suggesting that hhex mutants lack lymphatic precursors (Fig. 3a–e ). To confirm this result, we analyzed the TgBAC(prox1a:TagRFP) line which at 36 hpf labels lymphatic precursors prior to their migration from the PCV [20] . Imaging the trunk vasculature of hhex mutants at 36 hpf confirmed that the number of lymphatic precursors, as assessed by TagRFP expression, were strongly decreased compared to wild type (Fig. 3f–j ). Fig. 3 Zebrafish hhex mutants lack lymphatic precursors. a – d Whole-mount views of 36 hpf hhex +/+ and hhex −/− embryos immunostained for Prox1 (arrowheads point to Prox1 + endothelial cells in the PCV). e Quantification of the number of Prox1 + endothelial cells across three somites (from two field of view per embryo) in hhex +/? ( n = 8) and hhex −/− ( n = 6). f – i Whole-mount views of 36 hpf Tg(prox1a:TagRFP); hhex +/+ and hhex −/− embryos. hhex mutants exhibit a strong decrease in the number of RFP + cells in the PCV compared to hhex +/+ (arrowheads point to RFP + endothelial cells in the PCV). j Quantification of the number of RFP + endothelial cells across three somites (from two field of view per embryo) in hhex +/? ( n = 10) and hhex −/− ( n = 4). Values represent means ± s.e.m. *** P ≤ 0.001, and ** P ≤ 0.01 by t -test. Scale bars: 50 μm Full size image Cell-autonomous requirement for Hhex in sprouting angiogenesis Since hhex is expressed not only in endothelial cells but also in endodermal cells [5] , [22] and the endoderm has been shown to be important for sprouting angiogenesis from the PCV in zebrafish [23] , we sought to determine in which tissue(s) Hhex was required for angiogenesis. First, we performed whole-mount in situ hybridization for hhex expression at 36 hpf, when sprouting angiogenesis starts from the PCV, and at 48 hpf when vISVs have formed. At 36 hpf, hhex expression is enriched in budding endothelial cells in the PCV (Supplementary Fig. 3a ); in transverse sections, hhex expression is observed in the PCV and in the ventral wall of the dorsal aorta (Supplementary Fig. 3b ). At 48 hpf, hhex is expressed in vISVs and does not appear to be expressed in aISVs based on in situ analysis (Supplementary Fig. 3c ). These data indicate that hhex is expressed in endothelial cells during sprouting angiogenesis from the PCV. To determine whether Hhex regulates its own expression, we performed whole-mount in situ hybridization for hhex in hhex s722 mutants at 32 hpf. Interestingly, we observed that endothelial hhex expression was increased in hhex −/− compared to wild-type (Supplementary Fig. 4a, b ). To test whether the hhex s722 allele encodes a non-functional protein, we injected wild-type and mutant hhex mRNA into wild-type zebrafish embryos at the one-cell to four-cell stage (Supplementary Fig. 4c ). Overexpression of wild-type hhex led to strong developmental defects when injecting 50 to 200 pg while injection of similar amounts of hhex s722 mRNA had little effects on embryonic development (Supplementary Fig. 4c ). Altogether, these data indicate that the hhex s722 allele encodes a non-functional protein and that hhex can negatively regulate its own expression. To investigate the requirement of hhex in endothelial cells to form vISVs and LECs, we generated mosaic animals by transplanting wild-type Tg(fli1.ep:DsRedEx) donor cells into TgBAC(etv2:EGFP) hosts derived from hhex +/− incrosses. At 5 dpf, we imaged successfully transplanted larvae and quantified both vISV and TD extensions. We observed that transplanted wild-type endothelial cells were able to contribute to arteries, veins, and lymphatics in wild-type siblings as well as in mutant hosts (Fig. 4a, b and Supplementary Fig. 5 ). Indeed, transplanted wild-type cells could rescue both vISV and TD formation in hhex mutants (Fig. 4c, d ). Interestingly, wild-type and hhex mutant cells could be observed in vISVs, suggesting a defect in tip cell specification or behavior in hhex mutant cells. Wild-type tip cells may thus be sufficient to guide hhex mutant stalk cells and assemble a mosaic ISV. However, only wild-type cells were detectable in the TD of hhex mutants hosts, indicating that hhex is necessary for LEC differentiation. Fig. 4 Hhex is required cell-autonomously in endothelial cells to promote venous and lymphatic sprouting in zebrafish. a , b Transplantation of Tg(fli1ep:DsRedEx) donor cells into TgBAC(etv2:EGFP) hosts derived from hhex +/− incrosses. Wild-type endothelial cells contribute to arteries, veins, and lymphatics in wild-type sibling ( a ) and mutant ( b ) hosts at 5 dpf (arrowheads point to vISVs; asterisks indicate TD). c , d Quantification of vISVs ( c ) and TD extensions ( d ) across four somites in hhex −/− larvae with transplanted wild-type cells ( n = 13) vs. hhex −/− larvae without transplanted wild-type cells ( n = 6) at 5 dpf. Wild-type endothelial cells can partially rescue both vISV and TD formation in hhex −/− . e hhex endothelial overexpression strategy using the fli1a promoter partially rescues the hhex −/− vascular phenotype (arrowheads point to vISVs; asterisks indicate TD). f , g Quantification of vISVs ( f ) and TD ( g ) extensions across four somites in hhex −/− ( n = 6) and Tg(fli1a:tdTomato-2A-hhex); hhex −/− ( n = 6). h RNA sequencing of 48 hpf FACS-sorted hhex −/− endothelial cells and hhex -overexpressing endothelial cells. Heat map comparisons between these datasets identify Hhex as a regulator of genes implicated in lymphatic specification ( prox1a , prox1b , mafba , sox18 , nr2f2 ) and Flt4 signaling ( nrp2a , nrp2b , flt4 , vegfc ) while endothelial cell markers are modulated only by endothelial-specific hhex overexpression. Values represent means ± s.e.m. **** P ≤ 0.0001 and *** P ≤ 0.001 by t -test. Scale bars: 50 μm Full size image To further test the endothelial-autonomous requirement of Hhex in sprouting angiogenesis, we overexpressed hhex in endothelial cells using the fli1a promoter and visualized the transgenic cells by fusing tdTomato to the hhex coding sequence separated by a self-cleaving viral 2A peptide sequence (Fig. 4e ). We generated a stable transgenic line, Tg(fli1a:tdTomato-2A-hhex) , in which vascular and lymphatic development appeared to be unaffected (Supplementary Fig. 6 ) and crossed it to hhex +/− . Incrosses of Tg(fli1a:tdTomato-2A-hhex); hhex +/− were used to assess and quantify the rescue of the vascular phenotypes at 5 dpf. Quantification of vISV and TD extensions shows that hhex expression in endothelial cells was sufficient to rescue both vISV and TD network formation in hhex mutants (Fig. 4f, g ), thereby confirming the cell-autonomous function of Hhex during the formation of these structures identified in the cell transplantation experiments. To identify additional Hhex target genes, we performed RNA sequencing on 48 hpf hhex mutant endothelial cells, hhex -overexpressing endothelial cells, and wild-type endothelial cells (Fig. 4h ). Analysis of gene set enrichments between endothelial overexpression and mutant conditions pointed to a role for hhex in lymphatic vessel development (upregulation) and hematopoiesis (downregulation) (Supplementary Fig. 7a, b ), while comparisons between endothelial overexpression and wild-type conditions pointed to a role for hhex in vascular development (upregulation) and hematopoiesis (downregulation) (Supplementary Fig. 7c, d ). By comparing endothelial overexpression and mutant conditions, we also found that the expression of genes implicated in lymphatic specification ( prox1a , prox1b , sox18 , nr2f2 , mafba ) and Flt4 signaling ( nrp2a , nrp2b , flt4 ) was modulated by Hhex (Fig. 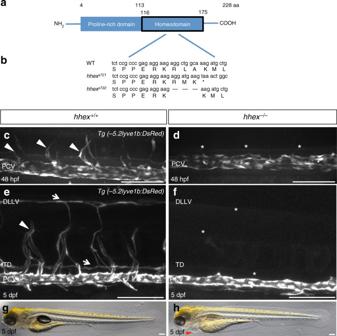Fig. 1 Zebrafishhhexmutants lack sprouting angiogenesis from the posterior cardinal vein.aSchematic representation of Hhex. Hhex, 228 amino acids (aa) long, is composed of a proline-rich domain (4–113 aa) and a homeodomain (116–175 aa).bAlignment of partial Hhex homeodomain sequence in wild-type (WT), and two mutant alleles,hhexs721andhhexs722. Thehhexs721allele contains a 10 bp insertion leading to a premature stop codon within the homeodomain coding region, whereas thehhexs722allele lacks amino acids R149 to A151.c,dTrunk vasculature ofTg(−5.2lyve1b:DsRed);hhex+/+andhhex−/−embryos at 48 hpf.hhexmutant trunks exhibit a defect in sprouting angiogenesis from the posterior cardinal vein (PCV) (arrowheads point to tip cells sprouting from the PCV; asterisks indicate lack of tip cells sprouting from the PCV).e,fTrunk vasculature ofTg(−5.2lyve1b:DsRed);hhex+/+andhhex−/−larvae at 5 dpf.hhexmutant trunks exhibit a defect in the formation of the venous intersegmental vessels (vISVs), the thoracic duct (TD) lymphatic vessel, and the dorsal longitudinal lymphatic vessel (DLLV) (arrowhead points to a vISV; arrows point to the ventrally positioned TD and dorsally positioned DLLV; asterisks indicate lack of these structures).g,hBrightfield lateral views ofhhex+/+andhhex−/−larvae at 5 dpf. Mutant larvae exhibit pericardial edema (arrowhead). Scale bars: 100 μm 4h and Supplementary Table 1 ). Interestingly, endothelial expression of sox18 and nr2f2 did not seem to be affected in hhex mutants but was upregulated following Hhex overexpression. The expression of venous markers including stab1 , stab2 , ephb4a , ephb4b , and mrc1a did not appear to be strongly modulated in hhex mutant endothelial cells, except for that of lyve1b . As Hhex expression has been shown to be enriched in tip cells [24] , we also checked different tip cell markers ( apln , aplnrb , adgrl4 , esm1 , igfbp3 , pfkfb3 ) and found that hhex overexpression enhanced aplnrb expression but decreased apln expression. Finally, using quantitative PCR (qPCR) analysis to further test the RNA sequencing data, we found that hhex could regulate vegfc , flt4 , and prox1a expression even though hhex overexpression was not sufficient to increase prox1a expression (Supplementary Fig. 7e ). Altogether, these data indicate that Hhex can cell-autonomously regulate the expression of genes implicated not only in lymphangiogenesis but also in sprouting angiogenesis. HHEX regulates angiogenesis and lymphangiogenesis in mammals To determine whether HHEX function in angiogenesis and lymphangiogenesis is conserved in mammals, we first took advantage of a previously described Hhex-IRES-Venus mouse reporter line [25] . We performed immunostaining on transverse sections from embryonic (E) day  E10.5 embryos focusing on the CV region where LEC precursors are still located within the vein and where specified LECs have already migrated outside the vein. We observed Hhex reporter expression in PECAM + blood endothelial cells as well as in PECAM + /PROX1 + LECs (Fig. 5a–d ). We also performed immunostaining on adult skin and small intestine and observed that the Hhex reporter is still expressed in blood endothelial cells and LECs (Fig. 5e–l ). These data show that the Hhex reporter is expressed by endothelial cells in both blood and lymphatic vessels, from early development until adulthood. Fig. 5 Hhex-IRES-Venus is expressed by vascular endothelial cells and lymphatic endothelial cells during mouse development and adulthood. a – d Maximum intensity projections of confocal images of an E10.5 Hhex-IRES-Venus embryo in the CV region after Venus (white), PROX1 (green), and PECAM (red) immunostaining. e – l Maximum intensity projections of confocal images of an Hhex-IRES-Venus adult mouse small intestine ( e – h ) and skin ( i – l ) after Venus (white), LYVE1 (blue) and PECAM (red) immunostaining. Hhex-IRES-Venus expression is observed in blood endothelial cells (red arrowheads) as well as LECs (white arrowheads). Scale bars: 50 μm Full size image To understand the precise function of Hhex during angiogenesis and lymphangiogenesis, we reanalyzed the phenotype of the global Hhex knockout by crossing Hhex floxed mice ( Hhex fl/fl ) [26] with Cmv-cre [27] to induce recombination in all tissues. We found that Hhex mutants were present at a Mendelian ratio at E10.5 and that this ratio decreased starting at E11.5 as previously described [8] . At E10.5, Hhex mutant mice exhibited pericardial edema and developmental delay (Supplementary Fig. 8a, b ). To characterize the vascular phenotype, we first performed whole-mount PECAM immunostaining on E10.5 embryos and observed strong vascular defects in the head and in the intersomitic vessels in the trunk (Supplementary Fig. 8c–f ). We also analyzed the CV region and found a decreased number of PROX1 + LECs within the CV and these cells appeared to exhibit weaker PROX1 immunostaining than in wild-types (Supplementary Fig. 8g–i ). At E14.5, only 12.5% of Hhex mutants could be recovered (mostly as dead or resorbed embryos), and the few surviving Hhex mutants presented strong vascular defects and blood-filled lymphatics (Supplementary Fig. 7j, k ). As the strong vascular defects we observed in Hhex mutants can affect the number of lymphatic precursors, we decided to cross Hhex fl/fl with Tie2-cre mice [28] which carry a cre transgene active in the blood islands at early stages and targeting both endothelial and hematopoietic cells [29] . No Tie2-cre Hhex fl/fl animals were recovered at birth, suggesting that mice lacking Hhex in Tie2 -expressing cells die during embryogenesis. At E10.5, Tie2-cre Hhex fl/fl embryos were recovered at a Mendelian ratio and, similarly to what was observed with the global Hhex mutants, this ratio decreased starting at E11.5. Tie2-cre Hhex fl/fl embryos exhibited pericardial edema and developmental delay (Fig. 6a ). Similarly, Flt4 mutant embryos started to die from E10.5 due to severe cardiovascular defects and exhibited yolk sac vasculature defects, pericardial edema, and developmental delay [30] . We performed whole-mount FLT4 immunostaining on E10.5 embryos and observed that Tie2-cre Hhex fl/fl embryos exhibited a strong decrease in FLT4 immunostaining notably in the intersomitic vessels (Fig. 6b, c ), possibly explaining the vascular phenotype. To further characterize the vascular phenotype, we also performed whole-mount PECAM immunostaining on E10.5 embryos and observed some vascular branching defects in the head (Fig. 6d–f ). Fig. 6 Tie2-cre Hhex fl/fl mouse embryos exhibit minor vascular defects and a reduced number of PROX1 + endothelial cells at E10.5. a Whole-mount view of Hhex fl/fl and Tie2-cre Hhex fl/fl embryos at E10.5. Hhex mutants exhibit pericardial edema (red arrowhead) as well as developmental delay. b , c Whole-mount views of Hhex fl/fl and Tie2-cre Hhex fl/fl embryos at E10.5 after FLT4 immunostaining. Hhex mutants exhibit a strong decrease in FLT4 expression in the intersomitic vessels (arrowheads point to intersomitic vessels; asterisks indicate reduction of FLT4 expression in the same structures). d – f Whole-mount view of Hhex fl/fl and Tie2-cre Hhex fl/fl embryos at E10.5 after PECAM immunostaining. Hhex mutants exhibit minor vascular defects in the head (arrowheads point to blood vessels in Hhex fl/fl and Tie2-cre Hhex fl/fl ; asterisk indicates lack of vessels in the same structures in Tie2-cre Hhex fl/fl ). g , h Maximum intensity projections of confocal images from transverse cryosections of Hhex fl/fl and Tie2-cre Hhex fl/fl E10.5 embryos after immunostaining for PECAM (white) and PROX1 (green) in the cardinal vein (CV) and aorta (A) region. Hhex mutants exhibit fewer PROX1 + /PECAM + endothelial cells in the region of the CV (arrowheads point to PROX1 + /PECAM + endothelial cells). i Quantification of the number of PROX1 + endothelial cells in the CV region in Hhex fl/fl ( n = 2) and Tie2-cre Hhex fl/fl ( n = 2) embryos. Values represent means ± s.e.m. ** P ≤ 0.01 by t -test. Scale bars: 1 mm ( a , d ), 200 μm ( b , c ), 500 μm ( e , f ), and 20 μm ( g , h ) Full size image The VEGFC/FLT4/PROX1 signaling axis has been shown to regulate the number of LECs in a dose-dependent manner [21] , [31] , [32] . To investigate whether HHEX affects the number of LECs, we quantified the number of PROX1 + cells in the CV region. Tie2-cre Hhex fl/fl mutants contained fewer PROX1 + endothelial cells in the CV compared to wild-type siblings (Fig. 6g–i ). Importantly, and as observed in global Hhex −/− embryos, these LECs were mostly within the vein and rarely outside. As decreased expression levels of Flt4 and Prox1 have been shown to trigger the same phenotype, these results suggest a migration defect in addition to the observed reduction in the number of LECs. At E14.5, the percentage of Tie2-cre Hhex fl/fl embryos recovered was below the expected Mendelian ratio (around 15% instead of the expected 25%), indicating that some Tie2-cre Hhex fl/fl embryos die at earlier stages. Tie2-cre Hhex fl/fl embryos alive at this stage exhibited severe lymphatic defects with edema and blood-filled lymphatics (Fig. 7a, c, e-f ). Moreover, whole-mount LYVE1 immunostaining revealed that Tie2-cre Hhex fl/fl embryos exhibit defects in the superficial lymphatic vasculature including a reduction in the number of lymphatic vessels (Fig. 7b, d ). We also examined the effects of deleting Hhex in Tie2-Cre -expressing cells on the blood and lymphatic vasculature using the dorsal skin model. At E14.5, LECs sprout and migrate towards the dorsal midline to form a stereotypical network [33] . Whole-mount immunostaining of the embryonic mouse skin with PECAM and NRP2 antibodies showed that both blood and lymphatic vascular networks were strongly affected in Tie2-cre Hhex fl/fl embryos compared to Hhex fl/fl (Fig. 7g–j ). Interestingly, lymphatic vessels in Tie2-cre Hhex fl/fl mutants displayed decreased intensity of NRP2 immunostaining compared to wild-type. Fig. 7 Tie2-cre Hhex fl/fl mouse embryos exhibit strong vascular and lymphatic defects at E14.5. a – c Morphology of Hhex fl/fl and Tie2-cre Hhex fl/fl mouse embryos at E14.5. Hhex inactivation in Tie2 -expressing cells leads to lymphatic defects including edema and blood-filled lymphatics (arrowheads). b – d Whole-mount views of Hhex fl/fl and Tie2-cre Hhex fl/fl embryos at E14.5 after LYVE1 immunostaining. Hhex mutants exhibit defects in lymphatic patterning with a reduced lymphatic vasculature in the skin (arrowheads indicate LYVE1 + lymphatic vessels, asterisks indicate lack of these vessels in the same area in Tie2-cre Hhex fl/fl ). e , f Brightfield pictures of Hhex fl/fl and Tie2-cre Hhex fl/fl skin at E14.5. Hhex mutants exhibit blood-filled lymphatics (arrowheads). g , h Whole-mount views of Hhex fl/fl and Tie2-cre Hhex fl/fl skin at E14.5 after PECAM immunostaining. Hhex mutants exhibit strong vascular defects at E14.5. i , j Whole-mount views of Hhex fl/fl and Tie2-cre Hhex fl/fl skin at E14.5 after NRP2 immunostaining. Hhex mutants exhibit strong lymphatic defects at E14.5 (arrows point to lymphatic vessels; arrowheads point to blood-filled lymphatic vessels with decreased intensity of NRP2 immunostaining). Scale bars: 2 mm ( a , c ), 1 mm ( b , d ), 200 μm ( e , f ), and 250 μm ( g – j ) Full size image In order to investigate the role of Hhex during lymphatic development, we crossed Hhex fl/fl with Prox1-cre ERT2 , a tamoxifen-inducible cre recombinase expressed in LECs [34] . Tamoxifen delivery from E10.5 to 12.5 to delete Hhex in LECs after their specification resulted in edema and blood-filled lymphatics at E16.5 (Fig. 8a–d ). Additionally, 10% of Prox1-cre ERT2 Hhex fl/fl embryos were found dead at this stage. Whole-mount immunostaining of the embryonic mouse skin with PECAM and NRP2 antibodies showed that the blood vascular network was not affected in Prox1-cre ERT2 Hhex fl/fl embryos, while the lymphatic network was clearly affected (Fig. 8e–h ). The lymphatic vessels were shorter, wider, and exhibited fewer branches in mutants compared to wild-types (Fig. 8i–k ). These results show that Hhex is important for the establishment of the lymphatic network during dermal lymphatic formation. Altogether, we investigated the role of Hhex during blood and lymphatic vascular development using global and conditional mouse mutants. The timing of Hhex recombination as well as the different phenotypes observed in Hhex −/− , Tie2-cre Hhex fl/fl , and Prox1-cre ERT2 Hhex fl/fl embryos are summarized in Fig. 9 . Fig. 8 Prox1-cre ERT2 Hhex fl/fl mouse embryos exhibit lymphatic defects at E16.5. a , b Whole-mount views of Hhex fl/fl and Prox1-cre ERT2 Hhex fl/fl embryos at E16.5 after tamoxifen injection at E10.5, 11.5, and 12.5. Hhex deletion in Prox1 -expressing cells leads to lymphatic defects including edema and blood-filled lymphatics (arrowheads). c , d Brightfield pictures of Hhex fl/fl and Prox1-cre ERT2 Hhex fl/fl skin at E16.5. Hhex mutants exhibit blood-filled lymphatics (arrowheads). e – h Whole-mount views of Hhex fl/fl and Prox1-cre ERT2 Hhex fl/fl skin at E16.5 after PECAM ( e – f ) and NRP2 ( g , h ) immunostaining. Hhex mutants do not exhibit vascular defects but clear lymphatic defects (arrowheads point to lymphatic vessels). i – k Quantification of the lymphatic network including average vessel width ( i ), average vessel length ( j ), and number of branch points (per mm vessel length) ( k ) in Hhex fl/fl ( n = 3) and Prox1-cre ERT2 Hhex fl/fl ( n = 3) skin at E16.5. Values represent means ± s.e.m. **** P ≤ 0.0001 and * P ≤ 0.05 by t -test. Scale bars: 1 mm ( a , b ), 200 μm ( c , d ), and 250 μm ( e – h ) Full size image Fig. 9 Summary of the effects of global and conditional Hhex deletion during vascular development in mouse. a Stages when Hhex recombination occurs in Hhex −/ − , Tie2-cre Hhex fl/fl , and Prox1-cre ERT2 Hhex fl/fl . b Consequences of Hhex deletion in Hhex -/- , Tie2-cre Hhex fl/fl , and Prox1-cre ERT2 Hhex fl/f are summarized in the blue boxes Full size image To test whether the role of HHEX is conserved in humans, we performed cell culture experiments to knockdown HHEX in human umbilical vein endothelial cells (HUVECs) (Fig. 10a ) and in human dermal LECs (HDLECs) (Fig. 10b ). Similarly to what we observed in both zebrafish and mouse embryos, decrease of HHEX expression in HUVECs and HDLECs led to decreased expression of FLT4 while VEGFC was upregulated (Fig. 10a, b ). Interestingly, HHEX knockdown in HDLECs also led to downregulation of PROX1 expression consistent with our observations in zebrafish and mouse (Fig. 10b ). Fig. 10 HHEX regulates the VEGFC/FLT4/PROX1 pathway in human endothelial cells and binds the PROX1 promoter. a , b qPCR analysis of HHEX , VEGFC , FLT4 , LYVE1 , PROX1 , and PECAM expression in HUVECs ( a ) and HDLECs ( b ) treated with HHEX siRNA compared to control cells treated with a scrambled siRNA. Knockdown of HHEX led to downregulation of FLT4 , PROX1 , and LYVE1 and upregulation of VEGFC expression. c Chromatin immunoprecipitation (ChIP) experiment using Myc-HHEX adenovirus in HUVECs. qPCR using primers for specific FLT4 , VEGFC , and PROX1 regions was carried out and enrichment relative to the percentage of input in the IP sample at PRM2 (control region) is shown. HHEX does not appear to bind the FLT4 promoter or VEGFC 3′ region but strongly binds the PROX1 promoter. Values represent means ± s.e.m. ** P ≤ 0.01; * P ≤ 0.05; ns, not significant by Mann-Whitney ( a , b ) or Bonferroni post hoc ( c ) Full size image Using in silico predictions, we identified putative HHEX binding sites 2 kb upstream of the FLT4 transcriptional start site, 800 bp upstream of the PROX1 transcriptional start site, and in the 3′ region of VEGFC . To test whether the transcriptional changes we observed were a result of direct HHEX binding to VEGFC , FLT4 , and PROX1 regulatory elements or via indirect routes, we performed chromatin immunoprecipitation (ChIP) experiments using Myc-HHEX adenovirus transfected in HUVECs (Fig. 10c ). We observed a significant enrichment of Myc-HHEX at the putative HHEX binding sites upstream of the PROX1 transcriptional start site (Fig. 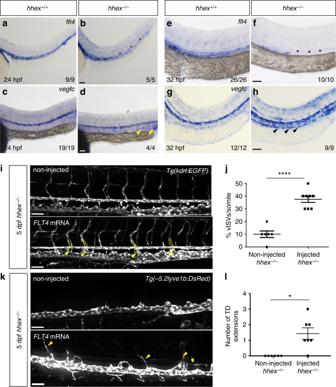Fig. 2 The Vegfc/Flt4 pathway is affected in zebrafishhhexmutants.a–dWhole-mount in situ hybridization showingflt4(a,b) andvegfc(c,d) expression in 24 hpfhhex+/+andhhex−/−embryos. At 24 hpf,hhexmutants exhibit decreasedflt4expression (asterisks), whereasvegfcexpression in the PCV appears to be slightly increased (arrowheads).e–hWhole-mount in situ hybridization showingflt4(e,f) andvegfc(g,h) expression at 32 hpf inhhex+/+andhhex−/−embryos. At 32 hpf,hhexmutants exhibit a strong decrease inflt4expression (asterisks), whereasvegfcexpression is clearly increased in the PCV (arrowheads).x/y: number of embryos showing representative phenotype (x), number of embryos examined (y).iTrunk vasculature of 5 dpfTg(kdrl:EGFP); hhex−/−injected, or not, with full-length humanFLT4mRNA.hhexmutants exhibit partial rescue of their vISVs at 5 dpf (arrowheads point to vISVs).jQuantification of vISVs across 10 somites in 5 dpf non-injectedhhex−/−(n= 6) andFLT4mRNA-injectedhhex−/−(n= 8).kTrunk lymphatic vasculature of 5 dpfTg(−5.2lyve1b:DsRed); hhex−/−injected, or not, with full-length humanFLT4mRNA.hhexmutants exhibit partial rescue of their TD at 5 dpf (arrowheads point to vISVs and arrow points to TD).lQuantification of TD extensions across 10 somites in 5 dpf non-injectedhhex−/−(n= 6) andFLT4mRNA-injectedhhex−/−(n= 7). Values represent means ± s.e.m. ****P≤ 0.0001 and *P≤ 0.05 byt-test. Scale bars: 50 μm 10c ), suggesting that PROX1 is a direct transcriptional target of HHEX. In contrast, our analyses did not show binding of HHEX directly to potential regulatory regions of FLT4 or VEGFC (Fig. 10c ), suggesting that HHEX regulation of these targets is indirect, or that other HHEX binding sites are present in distal regions. Altogether, these data indicate that HHEX regulates the VEGFC/FLT4/PROX1 axis in zebrafish, mouse, and human endothelial cells. Although the transcriptional networks underlying the development of the blood and lymphatic vessels have started to become better described, a complete understanding of these processes remains a major goal. Here, using a combination of systems and approaches, we have shown that the transcription factor HHEX functions upstream of several key players in blood and lymphatic vessel development, namely those of the VEGFC/FLT4/PROX1 axis. The formation of the lymphatic vasculature through the VEGFC/FLT4/PROX1 axis is an evolutionarily conserved process across vertebrates. Here, using zebrafish, we showed that hhex is necessary for venous and lymphatic sprouting from the PCV. hhex mRNA expression is not restricted to lymphatic precursors as marked by Prox1 expression, but is observed in both venous endothelial cells and LECs during sprouting from the PCV. hhex mutants exhibit unique gene expression changes, with a strong decrease in flt4 expression coupled to ectopic expression of vegfc in the PCV. 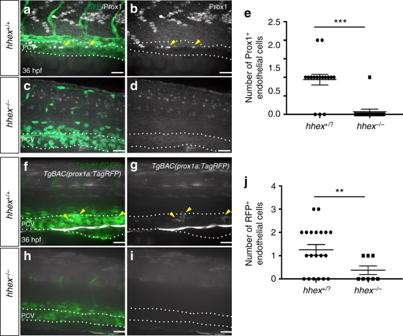Fig. 3 Zebrafishhhexmutants lack lymphatic precursors.a–dWhole-mount views of 36 hpfhhex+/+andhhex−/−embryos immunostained for Prox1 (arrowheads point to Prox1+endothelial cells in the PCV).eQuantification of the number of Prox1+endothelial cells across three somites (from two field of view per embryo) inhhex+/?(n= 8) andhhex−/−(n= 6).f–iWhole-mount views of 36 hpfTg(prox1a:TagRFP); hhex+/+andhhex−/−embryos.hhexmutants exhibit a strong decrease in the number of RFP+cells in the PCV compared tohhex+/+(arrowheads point to RFP+endothelial cells in the PCV).jQuantification of the number of RFP+endothelial cells across three somites (from two field of view per embryo) inhhex+/?(n= 10) andhhex−/−(n= 4). Values represent means ± s.e.m. ***P≤ 0.001, and **P≤ 0.01 byt-test. Scale bars: 50 μm Interestingly, FLT4 overexpression in zebrafish hhex mutants did not completely rescue the angiogenic defects. It is possible that the loss of hhex function affects additional pathways involved in sprouting angiogenesis from the vein, or that the FLT4 mRNA injections are not able to provide adequate levels of Flt4 function when needed. Furthermore, overexpression of hhex in endothelial cells increased flt4 expression while vegfc was downregulated. One possible explanation for these observations is that reduction of flt4 expression could affect vegfc expression and vice versa. However, Le Guen et al. [19] showed that flt4 level was not affected in vegfc morphants (and vice versa), thus indicating that Vegfc and Flt4 do not cross-regulate each other transcriptionally. Thus, Hhex appears to regulate at the same time and in an opposite fashion the transcription of genes encoding a growth factor and its receptor. HHEX has also been implicated in a number of human pathologies, with a crucial role in several types of cancer [35] , [36] . HHEX is overexpressed in human acute myeloid leukemia [35] , while in breast cancer HHEX functions as a suppressor of tumor growth and negatively regulates VEGFC [37] . Additionally, HHEX expression is upregulated in dermal LECs from type 2 diabetes patients, suggesting a potential lymphatic role for HHEX in pathological conditions [38] . Our RNA sequencing data suggest that Hhex can negatively regulate its own expression in endothelial cells. Using in situ hybridization, we indeed observed that endothelial hhex expression was increased in hhex mutants. This finding is consistent with a recent report in hematopoietic cells [39] . PROX1 is one of the key transcription factors driving the fate and specification of LECs in all vertebrates. We found that hhex mutants lack lymphatic precursors as assessed by Prox1 immunostaining and TgBAC(prox1a: TagRFP ) expression. Interestingly, PROX1 is expressed in many of the same tissues and developmental stages as HHEX, including hepatoblasts [22] . Here, we show that HHEX and PROX1 are co-expressed in developing LECs and that HHEX is necessary for PROX1 mRNA and protein expression. RNA sequencing data of endothelial cells from whole zebrafish embryos indicate that hhex overexpression does not increase prox1a expression, suggesting that Hhex co-factors present in subsets of endothelial cells might be necessary to drive prox1 expression. Hhex and Prox1 are also both expressed in endodermal tissues in zebrafish [40] and mouse [41] embryos, and it will be interesting to analyze in detail the expression pattern of these genes in wild-type and mutant animals to better understand how these genes regulate and maintain the differentiation of various cell types including LECs. Our data show that Hhex is required cell-autonomously in endothelial cells to promote venous and lymphatic sprouting. Using transplants to generate genetic mosaics, we found that tip cells in mutant hosts were always wild-type while hhex mutant cells could participate in vISV formation, suggesting that Flt4 signaling is not uniformly required for vISV formation but only for tip cell identity and behavior. This observation has also been reported in other sprouting angiogenesis contexts including Wnt signaling and brain angiogenesis [42] . Additionally, we observed that only wild-type cells could be found in the TD indicating a strict cell-autonomous requirement for Hhex in LEC formation in zebrafish. Using different mouse models, we show that Hhex is important for angiogenesis and lymphangiogenesis. Hhex −/− embryos exhibit severe developmental defects in blood and lymphatic vessel development while Hhex deletion in a more specific cell population using the Tie2-cre driver recapitulates the global knockout phenotype. We found that Tie2-cre Hhex fl/fl embryos exhibit a strong decrease in FLT4 immunostaining at E10.5, possibly explaining the vascular phenotypes. We also observed a reduced number of Prox1 + cells within the cardinal vein at E10.5, and these cells had not moved out of the vessel, thus also suggesting a migration defect. It has been shown in mouse that reducing Vegfc , Flt4 , or Prox1 function affects lymphatic development through a feedback loop that controls LEC precursor migration out of the vein [21] , [43] . Therefore, the reduced pool of lymphatic precursors we observed in Hhex mutants might be explained by the direct regulation of Prox1 by HHEX, while the migration defects might be due to the downregulation of Flt4 . Tie2-cre mice have been shown to recombine in endothelial and hematopoietic cells which could also explain the blood-filled lymphatic phenotype we observed at later stages. To identify the direct effects of Hhex on LECs and avoid early defects in vascular development, we used a specific lymphatic cre line ( Prox1-cre ERT2 ) and found that Hhex recombination caused defects in the formation of the lymphatics. Importantly, it has been reported that Prox1-cre ERT2 is most effective at late embryonic stages (from E12.5 in the skin) [44] , suggesting that the phenotype we observed in the skin is due to a late deletion of Hhex , and may explain why we observed LEC migration rather than specification defects. Determining the role of Hhex during early lymphangiogenesis will likely require the use of other cre lines in order to target earlier time points. Importantly, our work has identified HHEX as a crucial transcriptional regulator of lymphangiogenesis and provides new insights into the transcriptional regulation of lymphatic differentiation and homeostasis. Lymphedema, a dysfunction of lymphatic vessels, has a worldwide incidence of 300 million cases and almost half of the cases have a genetic origin [45] . Yet, only very few causative mutations have been identified in these patients, making the identification of new candidate genes or signaling pathways regulating lymphatic development a crucial research interest [46] . Notably, most of the genes implicated in lymphatic pathologies are associated with the VEGFC/FLT4/PROX1 axis, which is essential for lymphatic physiology not only during development [1] , [3] , [31] but also during tissue regeneration and cancer [47] . Therefore, the analysis of additional HHEX targets may help identify novel genetic causes of lymphedema, and also better modulate lymphatic vessels in various pathologies. Zebrafish husbandry and strains All zebrafish husbandry was performed under standard conditions in accordance with institutional (MPG) and national ethical and animal welfare guidelines. We used the following lines: TgBAC(etv2:EGFP) ci1 [48] , Tg(kdrl:NLS-mcherry) is4 [49] , Tg(kdrl:EGFP) s843 [50] , Tg(fli1a:nEGFP) y7 [51] , and Tg(fli1a.ep:DsRedEx) um13 [52] , TgBAC(prox1a:KalT4-UAS:uncTagRFP) nim5 [53] , and Tg(-5.2lyve1b:DsRed) nz101 [54] . All experiments were performed using the hhex s722 allele. Imaging Images were acquired using a Nikon SMZ25, a Zeiss Stereo Discovery V8, a Zeiss LSM780 confocal, or a Zeiss LSM800 confocal after embryo anesthesia with a low dose of tricaine and immobilization in 2% low-melting agarose in glass bottom petridishes (MatTek corporation). For time-lapse imaging, images were acquired using a Zeiss Cell Observer SD microscope. Embryos were mounted in 0.6% low-melting agarose and kept at 28 °C. Time-lapse images were recorded every 30 min. Facial lymphatics were measured using the ZEN software to determine the extent of formation of the different facial lymphatic vessels [55] , [56] . Generation of hhex mutants hhex mutants were generated by TALEN mutagenesis targeting exon 3. TALENs were assembled using the Golden Gate method [13] and 100 pg of total capped RNA per TALEN arm was injected into one-cell stage embryos. The following TAL effector domains RVDs were used: NI NG HD NG NN NG HD NG HD HD NN HD HD HD NN NI NN and HD NG HD NN HD NG NN NI NN HD NG NN HD NI NN HD NI NG HD NG. Both alleles were genotyped by high-resolution melt analysis of PCR products. The primer sequences can be found in Supplementary Data 1 . Quantifications Quantification of vISVs and TD extensions was performed across somites located above the yolk sac extension. FLT4 mRNA injections Full-length human wild-type FLT4 cloned into pCS2 plasmid [18] was linearized using Not I. FLT4 mRNA was then synthesized using a mMESSAGE mMACHINE SP6 Kit (Life Technologies) and purified using an RNA Clean and Concentrator Kit (Zymo Research). FLT4 mRNA was injected at 300 pg per embryo at the one-cell stage. Whole-mount in situ hybridization For whole-mount in situ hybridization [57] , embryos were fixed in 4% paraformaldehyde (PFA) overnight at 4 °C and subsequently dehydrated in methanol and stored at −20 °C until needed. In the first day, embryos were rehydrated to phosphate-buffered saline (PBS)/0.1% Tween-20 and then digested in 10 μg ml −1 proteinase K (Roche) followed by fixation in 4% PFA. Embryos were pre-incubated with hybridization buffer at 70 °C for 3 h and then incubated with digoxigenin (DIG)-labeled RNA antisense probes at 70 °C overnight. The next day, after washing, the embryos were incubated with alkaline phosphatase-conjugated anti-DIG antibody (Roche) at 4 °C overnight. The last day, after washing, the signal was visualized with NBT-BCIP staining solution (Roche). Primer sequences used to generate the probes for hhex , flt4 [58] , and vegfc [59] can be found in Supplementary Data 1 . Transplantation experiments Cells from Tg(fli1.ep:DsRedEx) wild-type donor embryos were transplanted at mid-blastula stages into host embryos derived from TgBAC(etv2:EGFP); hhex +/− heterozygous incrosses. Successfully transplanted embryos were selected and imaged at 5 dpf. Quantification of vISVs and TD extensions was performed across four somites above the yolk sac extension. Transgenesis To generate the Tg(fli1a:tdTomato-2A-hhex) bns136 line, tdTomato was fused to the hhex coding sequence separated by a self-cleaving viral 2A peptide sequence using Cold Fusion Technology (System Biosciences). To generate the line, 25 pg of Tol2 transposase mRNA and 25 pg of pTol2-fli1a:tdTomato-2A-hhex DNA were co-injected at the one-cell stage. The primers used for genotyping hhex mutants in the transgenic endothelial overexpression background can be found in Supplementary Data 1 . Quantification and statistical analysis No statistical methods were used to predetermine sample size. The experiments were not randomized. The investigators were not blinded to allocation during experiments or outcome assessment, except for the data shown in Figs. 2 – 4a, b . Representative images were selected from at least three independent experiments. Statistical analysis was performed using the GraphPad software. Values are presented as mean ± s.e.m. P values (* P ≤ 0.05, ** P ≤ 0.01, *** P ≤ 0.001, **** P ≤ 0.0001) were calculated using Student’s t -test except for the qPCR (Mann–Whitney nonparametric test) and ChIP (Bonferroni post hoc) experiments. Mouse strains All mice used were on a C57BL/6J background. The Hhex fl/fl [26] , Tie2-cre [28] , Prox1-cre ERT2 [34] , Cmv-cre [27] , and Hhex-IRES-Venus [25] mouse strains have been described. To generate Hhex +/− mice, Cmv-cre females were crossed with Hhex fl/fl males. Mice positive for Cmv-cre were then outcrossed with C57BL/6J mice to generate Hhex +/− mice. Deletion of the Hhex locus was confirmed by PCR [60] . To generate embryos, Hhex +/− males were crossed with Hhex +l− females. Tie2-cre Hhex fl/+ males were crossed with Hhex fl/fl females to generate embryos. The day of vaginal plug observation was considered as E0.5. Prox1-cre ERT2 animals were crossed with Hhex fl/fl to generate Prox1-cre ERT2 Hhex fl/fl . Cre-mediated recombination was induced at E10.5, 11.5, and 12.5 by intraperitoneal tamoxifen injection (2.5 mg/25 g at 20 mg ml −1 ). Embryos were harvested at E16.5 for analysis. All mouse experiments were conducted in accordance with institutional (MPG) and national ethical and animal welfare guidelines. Immunostaining To perform PROX1 immunostaining [23] , [61] , zebrafish embryos were fixed overnight in 4% PFA, washed in 100% methanol, incubated 1 h on ice in 3% H 2 O 2 in methanol, washed in 100% methanol, and stored at −20 °C. Samples were then permeabilized in wash buffer (PBS/0.1% Tween/0.1%Triton), blocked in 10% goat serum/1% bovine serum albumin in wash buffer overnight at 4 °C, and incubated with Prox1 antibody (1:100, 102-PA32, Reliatech) overnight at 4 °C. Samples were then washed five times with wash buffer, followed by washes with maleic buffer (150 mM maleic acid/100 mM NaCl/0.001% Tween-20 pH 7.4), followed by blocking in maleic buffer containing 2% blocking reagent (Roche) for 3 h at room temperature, then incubated overnight at 4 °C with goat anti-rabbit IgG–horseradish peroxidase (Abcam, ab6721, 1:1000) for TSA signal amplification. Following washes with maleic buffer and PBS, samples were incubated for 3 h with TSA Plus Cyanine 5 reaction (Perkin Elmer) and washed with wash buffer several times over 1–2 days at room temperature. To perform whole-mount immunostaining in mouse [62] , tissues were fixed overnight in 4% PFA and blocked overnight in blocking buffer (TSA blocking reagent, Perkin Elmer). Tissues were then incubated for 2 days at 4 °C with biotinylated antibodies in blocking buffer followed by biotin-streptavidin-horseradish peroxidase amplifications using the Vectastain-ABC Kit (Vector labs). For cryostat sections, E10.5 embryos were fixed overnight in 4% PFA, cryopreserved with 30% sucrose before immersion in OCT (Tissue-Tek), and stored at −80 °C. Ten micrometer sections were selected (between the eyes and the heart) to identify the bilateral cardinal veins and perform quantification of LECs. For the analysis of the dorsal dermal lymphatic network, E16.5 embryos were fixed for 2 h in 4% PFA before the dorsal skin was dissected and stained. Quantification of skin lymphatic vessels was performed using ImageJ. The antibodies used were PECAM-1 (1:100, MEC13.3, BD Biosciences), GFP (1:100, GFP-1020, Aves Labs), LYVE1 (1:100, 103-PA50, Reliatech), FLT4 (1:100, AF743, R&D Systems), and NRP2 (1:100, AF567, R&D Systems). Primary cells HUVECs and HDLECs were obtained from Lonza, cultured with endothelial growth medium-2 (Lonza), and confluent cells were used at passage 6 or less. qPCR analysis of HUVECs showed very minimal expression of PROX1 , LYVE1 , and PDPN . siRNA-mediated knockdown Cells were transfected with small interfering RNAs (siRNAs) using Opti-MEM and Lipofectamine RNAiMAX (Invitrogen) [63] . The target sequence of the two siRNAs directed against HHEX mRNA can be found in Supplementary Data 1 . FACS sorting and RNA sequencing For isolating endothelial cells from 48 hpf Tg(kdrl:EGFP) siblings and hhex mutants, embryos were selected based on the presence or absence of parachordal lymphangioblasts. Embryos were then rinsed in HBSS (Gibco) followed by dissociation in TrypLE express (Gibco) at 28 °C with repeated pipetting. Endothelial cells were isolated using a BD Aria sorter and sorted for EGFP + or EGFP + /tdTomato + signals (for Tg(kdrl:EGFP ); Tg(fli1a:tdTomato-2A-hhex)) . RNA was isolated using the miRNeasy Micro Kit (Qiagen) combined with on-column DNase digestion (DNase-Free DNase Set, Qiagen) to avoid contamination by genomic DNA. RNA and library preparation integrity were verified with BioAnalyzer 2100 (Agilent) and LabChip Gx Touch 24 (Perkin Elmer). 6 ng of total RNA was used as input for SMARTer ® Stranded Total RNA-Seq Kit–Pico Input Mammalian Kit (Clontech). Sequencing was performed on a NextSeq500 instrument (Illumina) using v2 chemistry, resulting in a minimum of 30M reads per library with 1 × 75 bp single end setup. The resulting raw reads were assessed for quality, adapter content, and duplication rates with FastQC (Andrews S. 2010, FastQC: a quality control tool for high-throughput sequence data, http://www.bioinformatics.babraham.ac.uk/projects/fastqc ). Reaper version 13–100 was used to trim reads after a quality drop below a mean of Q20 in a window of 10 nucleotides [64] . Only reads between 30 and 150 nucleotides were cleared for further analyses. Trimmed and filtered reads were aligned vs. the zebrafish genome version DanRer10 (GRCz10.87) using STAR 2.4.0a with the parameter “--outFilterMismatchNoverLmax 0.1” to increase the maximum ratio of mismatches to mapped length to 10% [65] . The number of reads aligning to genes was counted with featureCounts 1.4.5-p1 tool from the Subread package [66] . Only reads mapping at least partially inside exons were admitted and aggregated per gene. Reads overlapping multiple genes or aligning to multiple regions were excluded. Differentially expressed genes were identified using DESeq2 version 1.62 [67] . Only genes with a maximum Benjamini–Hochberg corrected p value of 0.05, and a minimum combined mean of five reads were deemed to be significantly differentially expressed. The Ensemble annotation was enriched with UniProt data (release 06.06.2014) based on Ensembl gene identifiers. 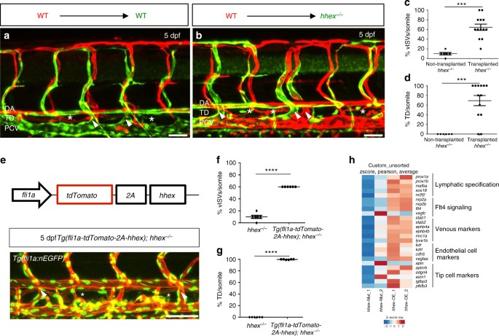Fig. 4 Hhex is required cell-autonomously in endothelial cells to promote venous and lymphatic sprouting in zebrafish.a,bTransplantation ofTg(fli1ep:DsRedEx)donor cells intoTgBAC(etv2:EGFP)hosts derived fromhhex+/−incrosses. Wild-type endothelial cells contribute to arteries, veins, and lymphatics in wild-type sibling (a) and mutant (b) hosts at 5 dpf (arrowheads point to vISVs; asterisks indicate TD).c,dQuantification of vISVs (c) and TD extensions (d) across four somites inhhex−/−larvae with transplanted wild-type cells (n= 13) vs.hhex−/−larvae without transplanted wild-type cells (n= 6) at 5 dpf. Wild-type endothelial cells can partially rescue both vISV and TD formation inhhex−/−.ehhexendothelial overexpression strategy using thefli1apromoter partially rescues thehhex−/−vascular phenotype (arrowheads point to vISVs; asterisks indicate TD).f,gQuantification of vISVs (f) and TD (g) extensions across four somites inhhex−/−(n= 6) andTg(fli1a:tdTomato-2A-hhex); hhex−/−(n= 6).hRNA sequencing of 48 hpf FACS-sortedhhex−/−endothelial cells andhhex-overexpressing endothelial cells. Heat map comparisons between these datasets identify Hhex as a regulator of genes implicated in lymphatic specification (prox1a,prox1b,mafba,sox18,nr2f2) and Flt4 signaling (nrp2a,nrp2b,flt4,vegfc) while endothelial cell markers are modulated only by endothelial-specifichhexoverexpression. Values represent means ± s.e.m. ****P≤ 0.0001 and ***P≤ 0.001 byt-test. Scale bars: 50 μm The gene set enrichment analysis was performed using Metascape [68] ( www.metascape.org ). The RNA-seq data can be accessed via the accession code GSE111963 ( https://www.ncbi.nlm.nih.gov/geo/query/acc.cgi?acc = GSE111963 ). 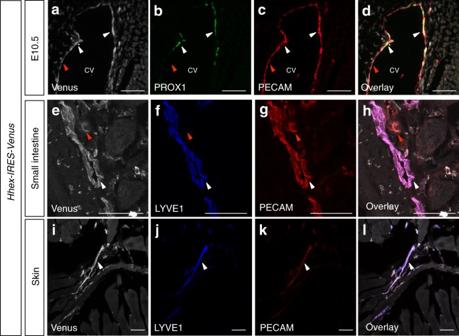Fig. 5 Hhex-IRES-Venusis expressed by vascular endothelial cells and lymphatic endothelial cells during mouse development and adulthood.a–dMaximum intensity projections of confocal images of an E10.5Hhex-IRES-Venusembryo in the CV region after Venus (white), PROX1 (green), and PECAM (red) immunostaining.e–lMaximum intensity projections of confocal images of anHhex-IRES-Venusadult mouse small intestine (e–h) and skin (i–l) after Venus (white), LYVE1 (blue) and PECAM (red) immunostaining.Hhex-IRES-Venusexpression is observed in blood endothelial cells (red arrowheads) as well as LECs (white arrowheads). Scale bars: 50 μm Validation of modulated genes was performed by qPCR on dissected trunks in hhex mutants, wild-type siblings, and Tg(fli1a:tdTomato-2A-hhex) embryos. Quantitative PCR Total RNA was isolated using the RNA Micro Kit (Qiagen). RNA was reverse transcribed using the Transcriptor High Fidelity cDNA Synthesis Kit (Roche) according to the manufacturer’s instructions. qPCR reactions were carried out using TaqMan Probe Master or SYBR Green I Master (Roche). Primer sequences used in this study are provided in Supplementary Data 1 . Chromatin immunoprecipitation HUVECs (5 × 10 6 cells per ChIP) were infected with Adenovirus Myc-HHEX or Adenovirus GFP control virus and ChIP experiments were done [69] using a Myc antibody (CST #9B11, 3 μg/ChIP). qPCR was performed in quadruplicate. All data were normalized to PRM2 (control). The control region used is located in chromosome 18 where HHEX should not bind. Primers used can be found in Supplementary Data 1 . 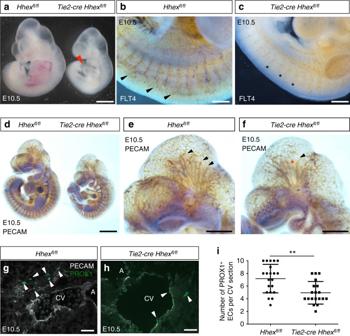Fig. 6 Tie2-cre Hhexfl/flmouse embryos exhibit minor vascular defects and a reduced number of PROX1+endothelial cells at E10.5.aWhole-mount view ofHhexfl/flandTie2-cre Hhexfl/flembryos at E10.5.Hhexmutants exhibit pericardial edema (red arrowhead) as well as developmental delay.b,cWhole-mount views ofHhexfl/flandTie2-cre Hhexfl/flembryos at E10.5 after FLT4 immunostaining.Hhexmutants exhibit a strong decrease in FLT4 expression in the intersomitic vessels (arrowheads point to intersomitic vessels; asterisks indicate reduction of FLT4 expression in the same structures).d–fWhole-mount view ofHhexfl/flandTie2-cre Hhexfl/flembryos at E10.5 after PECAM immunostaining.Hhexmutants exhibit minor vascular defects in the head (arrowheads point to blood vessels inHhexfl/flandTie2-cre Hhexfl/fl; asterisk indicates lack of vessels in the same structures inTie2-cre Hhexfl/fl).g,hMaximum intensity projections of confocal images from transverse cryosections ofHhexfl/flandTie2-cre Hhexfl/flE10.5 embryos after immunostaining for PECAM (white) and PROX1 (green) in the cardinal vein (CV) and aorta (A) region.Hhexmutants exhibit fewer PROX1+/PECAM+endothelial cells in the region of the CV (arrowheads point to PROX1+/PECAM+endothelial cells).iQuantification of the number of PROX1+endothelial cells in the CV region inHhexfl/fl(n= 2) andTie2-cre Hhexfl/fl(n= 2) embryos. Values represent means ± s.e.m. **P≤ 0.01 byt-test. Scale bars: 1 mm (a,d), 200 μm (b,c), 500 μm (e,f), and 20 μm (g,h) Data availability The authors declare that all data supporting the findings of this study are available within the article and its supplementary information files or from the corresponding authors upon reasonable request. 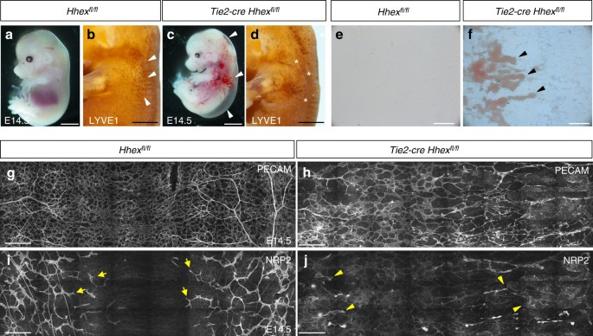Fig. 7 Tie2-cre Hhexfl/flmouse embryos exhibit strong vascular and lymphatic defects at E14.5.a–cMorphology ofHhexfl/flandTie2-cre Hhexfl/flmouse embryos at E14.5.Hhexinactivation inTie2-expressing cells leads to lymphatic defects including edema and blood-filled lymphatics (arrowheads).b–dWhole-mount views ofHhexfl/flandTie2-cre Hhexfl/flembryos at E14.5 after LYVE1 immunostaining.Hhexmutants exhibit defects in lymphatic patterning with a reduced lymphatic vasculature in the skin (arrowheads indicate LYVE1+lymphatic vessels, asterisks indicate lack of these vessels in the same area inTie2-cre Hhexfl/fl).e,fBrightfield pictures ofHhexfl/flandTie2-cre Hhexfl/flskin at E14.5.Hhexmutants exhibit blood-filled lymphatics (arrowheads).g,hWhole-mount views ofHhexfl/flandTie2-cre Hhexfl/flskin at E14.5 after PECAM immunostaining.Hhexmutants exhibit strong vascular defects at E14.5.i,jWhole-mount views ofHhexfl/flandTie2-cre Hhexfl/flskin at E14.5 after NRP2 immunostaining.Hhexmutants exhibit strong lymphatic defects at E14.5 (arrows point to lymphatic vessels; arrowheads point to blood-filled lymphatic vessels with decreased intensity of NRP2 immunostaining). Scale bars: 2 mm (a,c), 1 mm (b,d), 200 μm (e,f), and 250 μm (g–j) 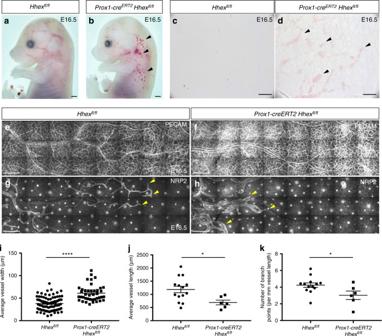Fig. 8 Prox1-creERT2Hhexfl/flmouse embryos exhibit lymphatic defects at E16.5.a,bWhole-mount views ofHhexfl/flandProx1-creERT2Hhexfl/flembryos at E16.5 after tamoxifen injection at E10.5, 11.5, and 12.5.Hhexdeletion inProx1-expressing cells leads to lymphatic defects including edema and blood-filled lymphatics (arrowheads).c,dBrightfield pictures ofHhexfl/flandProx1-creERT2Hhexfl/flskin at E16.5.Hhexmutants exhibit blood-filled lymphatics (arrowheads).e–hWhole-mount views ofHhexfl/flandProx1-creERT2Hhexfl/flskin at E16.5 after PECAM (e–f) and NRP2 (g,h) immunostaining.Hhexmutants do not exhibit vascular defects but clear lymphatic defects (arrowheads point to lymphatic vessels).i–kQuantification of the lymphatic network including average vessel width (i), average vessel length (j), and number of branch points (per mm vessel length) (k) inHhexfl/fl(n= 3) andProx1-creERT2Hhexfl/fl(n= 3) skin at E16.5. Values represent means ± s.e.m. ****P≤ 0.0001 and *P≤ 0.05 byt-test. Scale bars: 1 mm (a,b), 200 μm (c,d), and 250 μm (e–h) 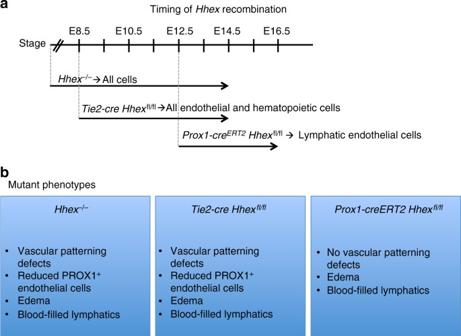Fig. 9 Summary of the effects of global and conditionalHhexdeletion during vascular development in mouse.aStages whenHhexrecombination occurs inHhex−/−,Tie2-cre Hhexfl/fl, andProx1-creERT2Hhexfl/fl.bConsequences ofHhexdeletion inHhex-/-,Tie2-cre Hhexfl/fl, andProx1-creERT2Hhexfl/fare summarized in the blue boxes 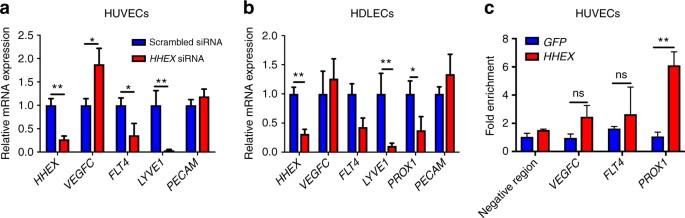Fig. 10 HHEX regulates the VEGFC/FLT4/PROX1 pathway in human endothelial cells and binds the PROX1 promoter.a,bqPCR analysis ofHHEX,VEGFC,FLT4,LYVE1,PROX1, andPECAMexpression in HUVECs (a) and HDLECs (b) treated withHHEXsiRNA compared to control cells treated with a scrambled siRNA. Knockdown ofHHEXled to downregulation ofFLT4,PROX1, andLYVE1and upregulation ofVEGFCexpression.cChromatin immunoprecipitation (ChIP) experiment usingMyc-HHEXadenovirus in HUVECs. qPCR using primers for specificFLT4,VEGFC, andPROX1regions was carried out and enrichment relative to the percentage of input in the IP sample atPRM2(control region) is shown. HHEX does not appear to bind theFLT4promoter orVEGFC3′ region but strongly binds thePROX1promoter. Values represent means ± s.e.m. **P≤ 0.01; *P≤ 0.05; ns, not significant by Mann-Whitney (a,b) or Bonferroni post hoc (c) The RNA-seq data have been deposited in the NCBI’s Gene Expression Omnibus database under accession code GSE111963 .